Involvement of parental imprinting in the antisense regulation of onco-miR-372-373 The monoallelic nature of imprinted genes renders them highly susceptible to genetic and epigenetic perturbations, potentially resulting in transformation and disease. Here we show, using parthenogenetic induced pluripotent stem cells, an imprinted transcript that serves as an antisense regulator of onco-miR-372-3 (named anti-miR-371-3). As miR-372-3 have been shown to have an oncogenic role in testicular germ cell tumours, we study the involvement of their antisense transcript in these cells. Our results suggest that hypermethylation, leading to loss-of-expression of the imprinted antisense transcript, contributes to tumorigenic transformation by affecting the downstream target LATS2 . Finally, we provide evidence for a tumour suppressive role of anti-miR-371-3, as its overexpression in tumour cells results in cell growth arrest and apoptosis, and prevents tumour formation on injection into immunodeficient mice. Parental imprinting is a form of parent-of-origin epigenetic marking inherited from the gametes [1] , which restricts asexual reproduction in placental mammals [2] , [3] . In humans, both complete maternal (parthenogenetic) and complete paternal (androgenetic) uniparental disomies result in different types of tumours [4] . While parthenogenesis generates ovarian teratomas, androgenesis leads to hydatidiform moles, a more aggressive and malignant form of tumours. These observations, along with the intrinsic monoallelic nature of imprinting, suggest that some imprinted genes may hold tumorigenic potential [5] . Indeed, loss-of-imprinting of several genes (for example, H19 , IGF2 and MEST ) has been correlated with different types of malignancies such as Wilm’s tumour [6] , colorectal neoplasia [7] and lung cancer [8] . Nevertheless, the causative role of imprinting in tumorigenesis is still poorly understood, and the precise mechanisms by which imprinted genes may contribute to tumorigenicity remain to be elucidated. Here we report the identification of a paternally expressed transcript, transcribed in the antisense orientation to the previously recognized oncogenic microRNA-372-373 (miR-372-3) cluster [9] . Further, we demonstrate that this antisense transcript may have a tumour suppressive role in testicular germ cell tumours (TGCTs) by regulating the expression of the corresponding miRs. Our data suggest that loss-of-imprinting in TGCTs contributes to the tumorigenicity of the cells by activating onco-miRs and promoting cell proliferation. An imprinted gene transcribed antisense to miR-371-3 Human parthenogenetic pluripotent stem cells (PSCs) lack the paternal genome and are thus considered a valuable tool in studying the role of parental imprinting during early human embryogenesis [10] . In these cells, paternally expressed genes (PEGs) are predicted to appear markedly downregulated when compared with normal bi-parental cells. Indeed, gene expression analysis in parthenogenetic human-induced PSCs (PgHiPSCs) has previously enabled us to identify both known and novel PEGs throughout the human genome [10] . Contrary to PEGs, maternally expressed genes are less easily identified using parthenogenetic cells, as they are expected to exhibit only a twofold increase compared with normal cells. Surprisingly, a comparison of miR expression data in parthenogenetic and normal cells revealed a pronounced overexpression of miR-371, miR-372 and miR-373 (miR-371-3) in PgHiPSCs relative to normal PSCs, including both human embryonic stem cells (HESCs) and induced PSCs (HiPSCs, Fig. 1a,b and Supplementary Data 1 ). This upregulation of miR-371-3 suggested that this cluster is either directly or indirectly regulated by PEGs. To uncover the mechanism controlling miR-371-3 expression, we performed strand-specific high-throughput RNA sequencing in two independent PgHiPSC lines and two control wild-type (WT) HESC and HiPSC lines. Interestingly, analysis of reads that mapped to the miR-371-3 region led to the identification of a putative gene, transcribed in the antisense orientation to the corresponding miRs, which we named anti-miR-371-3 ( Supplementary Fig. S1a ). In support of these findings, previously reported expressed sequence tags, pooled from normal testis tissue and germ cell tumours, verify transcription from both strands in this region ( Supplementary Fig. S1b ). Further, reads that mapped to the antisense strand may potentially mark a putative transcription start site of anti-miR371-3 ( Supplementary Fig. S1b ). Next, we quantified the ratios in reads per kilobase per million mapped reads (RPKM) for both strands, demonstrating that whereas miR-371-3 is upregulated in parthenogenetic cells, anti-miR-371-3 is significantly downregulated compared with normal PSCs ( Fig. 1c and Supplementary Fig. S1a ). The downregulation of anti-miR-371-3 observed in PgHiPSCs implicated it as a potential novel PEG. To examine this possibility, we utilized an informative single nucleotide polymorphism in the genomic region of anti-miR-371-3. By applying strand-specific RT–PCR and direct sequencing to two independent WT-PSC lines, we found monoallelic expression of the antisense strand at the RNA level ( Fig. 1d , Fig. 3d and Supplementary Fig. S1b,c ). However, application of the same method to the positive stand revealed biallelic expression of miR-371-3 ( Fig. 1d ). Taken together, our data imply that anti-miR-371-3 is a novel imprinted gene, expressed exclusively from the paternal allele, whereas miR-371-3 seems to be transcribed from both alleles in PSCs ( Fig. 1e ). To study the expression patterns of anti-miR-371-3 in other cell types representative of early human embryogenesis, we analysed its expression in 7-, 20- and 30-day-old embryoid bodies (EBs), in normal PSCs treated with BMP4 for 7 days (representing the trophectoderm lineage), in neural progenitor cells differentiated from normal PSCs (representing early neural differentiation) and in normal fibroblasts. This analysis identified downregulation of anti-miR-371-3 on in vitro differentiation in all cell types tested ( Fig. 1f,g ), suggesting that similar to the miR-371-3 cluster [11] , [12] , it is abundantly and predominantly expressed in PSCs. 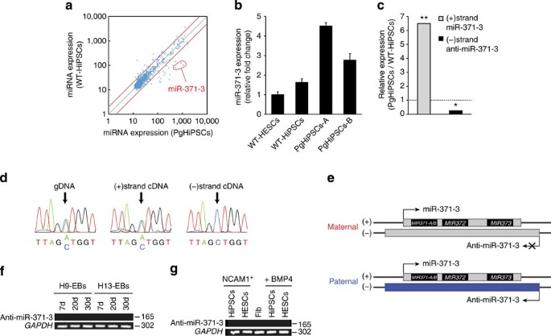Figure 1: Identification of an imprinted gene transcribed in the antisense orientation to miR-371-3. (a) Scatter-plot analysis comparing global microRNA expression between parthenogenetic and WT-PSCs (PgHiPSCs and WT-HiPSCs, respectively). Values are displayed on a logarithmic scale. (b) Expression of miR-371-3 by qRT–PCR. Shown are the relative expression levels of miR-371-3 (mean±s.d.) in four normal PSCs (both embryonic and induced PSCs) and four PgHiPSCs lines (two from each patient, represented as A and B). (c) Quantification of deep RNA sequencing analysis of the miR-371-3 locus in RPKM in two WT-PSC lines and two PgHiPSC lines, showing the relative expression of miR-371-3 (s.d.=0.028) and anti-miR-371-3 (s.d.=0.007) in PgHiPSCs versus normal PSCs. *P<0.05, **P<10−8, Cufflinks statistical test. (d) Sequencing of the transcribed region overlapping both miR-371-3 and anti-miR-371-3 in genomic DNA (gDNA) and strand-specific complementary DNA (cDNA) in normal HiPSCs. Note that anti-miR-371-3 is expressed only from one allele, whereas expression of miR-371-3 is biallelic. (e) Schematic genomic organization of miR-371-3 and its novel antisense transcript in the maternally and paternally inherited chromosomes. Blue box, PEG. (f) Expression patterns of anti-miR-371-3 as measured by strand-specific RT-PCR in 7-, 20- and 30-day-old EBs in two normal pluripotent cell lines. Band sizes are designated in bp. (g) Expression patterns of anti-miR-371-3 as measured by strand-specific RT-PCR in normal PSCs differentiated to neural progenitor cells and sorted for NCAM1-positive cells (Methods), normal fibroblasts and PSCs differentiated to trophectoderm-like cells by treatment with BMP4 for 7 days (Methods), Band sizes are designated in bp. Figure 1: Identification of an imprinted gene transcribed in the antisense orientation to miR-371-3. ( a ) Scatter-plot analysis comparing global microRNA expression between parthenogenetic and WT-PSCs (PgHiPSCs and WT-HiPSCs, respectively). Values are displayed on a logarithmic scale. ( b ) Expression of miR-371-3 by qRT–PCR. Shown are the relative expression levels of miR-371-3 (mean±s.d.) in four normal PSCs (both embryonic and induced PSCs) and four PgHiPSCs lines (two from each patient, represented as A and B). ( c ) Quantification of deep RNA sequencing analysis of the miR-371-3 locus in RPKM in two WT-PSC lines and two PgHiPSC lines, showing the relative expression of miR-371-3 (s.d.=0.028) and anti-miR-371-3 (s.d.=0.007) in PgHiPSCs versus normal PSCs. * P <0.05, ** P <10 −8 , Cufflinks statistical test. ( d ) Sequencing of the transcribed region overlapping both miR-371-3 and anti-miR-371-3 in genomic DNA (gDNA) and strand-specific complementary DNA (cDNA) in normal HiPSCs. Note that anti-miR-371-3 is expressed only from one allele, whereas expression of miR-371-3 is biallelic. ( e ) Schematic genomic organization of miR-371-3 and its novel antisense transcript in the maternally and paternally inherited chromosomes. Blue box, PEG. ( f ) Expression patterns of anti-miR-371-3 as measured by strand-specific RT-PCR in 7-, 20- and 30-day-old EBs in two normal pluripotent cell lines. Band sizes are designated in bp. ( g ) Expression patterns of anti-miR-371-3 as measured by strand-specific RT-PCR in normal PSCs differentiated to neural progenitor cells and sorted for NCAM1-positive cells (Methods), normal fibroblasts and PSCs differentiated to trophectoderm-like cells by treatment with BMP4 for 7 days (Methods), Band sizes are designated in bp. Full size image DNA methylation analysis at the miR-371-3 locus DNA methylation is considered as the hallmark mechanism regulating parental imprinting [13] . Imprinted differentially methylated regions (DMRs) are established in the germ cells and maintained throughout the development of the embryo, consequently regulating the monoallelic expression of imprinted genes, in all tissues or in a tissue-specific manner [14] . To study the DNA methylation signature at the miR-371-3 locus and nearby sequences, we employed our recently established genome-wide DNA methylation sequencing data from PgHiPSCs, multiple normal PSCs and somatic cells [15] . As our PgHiPSCs comprise a completely maternal diploid genome, we had been able to show that their DNA methylation pattern differs from that of normal PSCs in virtually all known imprinted DMRs [15] . We thus searched for novel DMRs adjacent to the miR-371-3 and anti-miR-371-3 genes. Hypermethylation of the miR-371-3 promoter was observed in all cell types tested, without any apparent differential DNA methylation upstream to anti-miR-371-3 ( Fig. 2a,b ). These results suggested that similar to many other imprinted genes, anti-miR-371-3 may be regulated in cis by a distant-imprinted DMR [1] , [16] . The miR-371-3 locus resides in proximity to the large miRs cluster C19MC, previously shown to be expressed exclusively from the paternal allele in the placenta [17] ( Fig. 2a ). Further upstream resides another putative imprinted gene called ZNF331 (refs 18 , 19 ) ( Fig. 2a ). Importantly, two putative maternal DMRs were identified in this locus; one upstream to C19MC and another upstream to ZNF331 ( Fig. 2a,b ). In agreement with previous findings in other tissues [17] , the C19MC DMR exhibits hypermethylation in both normal and parthenogenetic PSCs, correlating with lack of expression of C19MC in PSCs ( Fig. 2a–c ). Nevertheless, significant differences in DNA methylation were detected between parthenogenetic and normal cells in the DMR upstream to ZNF331 ( Fig. 2a,b ). Whereas undifferentiated and somatic WT cells show intermediate methylation values (mean methylation calls of 0.4–0.6), both PgHiPSCs and their parental fibroblasts show hypermethylation (mean methylation calls >0.6), thereby supporting the conclusion that the ZNF331 DMR is a maternally derived imprinted DMR ( Fig. 2a,b ). Next, we searched for imprinted DMRs in the promoters of other genes in the locus (secondary DMRs). No additional putative imprinted DMRs were found, correlating with no apparent differences in gene expression between parthenogenetic and normal PSCs ( Fig. 2a,b,d ). Taken together, our analysis of DNA methylation in the miR-371-3 locus confirmed the previously suggested imprinted DMR upstream to ZNF331 , which may also underlie the monoallelic expression of anti-miR-371-3 in PSCs. Notably, although this analysis covers the vast majority of CpG islands in the human genome, it only moderately represents low-density CpG regions. Therefore, it remains to be elucidated whether an imprinting-specific DMR exists in the promoters of miR-371-3 or anti-miR-371-3, or in another CpG-poor region adjacent to them. 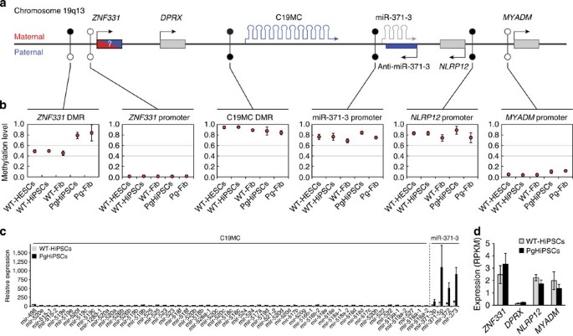Figure 2: DNA methylation and gene expression analyses at the miR-371-3 locus. (a) Schematic representation of the maternal and paternal genomic regions in which the miR-371-3 locus resides. Filled circle: methylated allele; empty circle: unmethylated allele. Maternally expressed genes and PEGs are designated in red and blue, respectively. Genes with biallelic expression are shown in grey. Note that current data regarding the parental expression ofZNF331are conflicting. (b) Mean methylation calls±s.d. across the region in different cell types; WT-HESCs (n=20), WT-HiPSCs (n=12), WT-Fib (n=6), PgHiPSCs (n=4) and Pg-Fib (n=2). DNA methylation levels (y-axis) vary between 0 (unmethylated) and 1 (fully methylated); 0.4–0.6, intermediate methylation values. (c) Expression levels (mean±s.d., in two WT-PSC lines and three PgHiPSC lines) of all annotated miRs in the region in WT-HiPSCs and PgHiPSCs. (d) Expression levels (mean±s.d., in two WT-PSC lines and two PgHiPSC lines) of annotated genes within the region, as determined by RNA sequencing analysis. Figure 2: DNA methylation and gene expression analyses at the miR-371-3 locus. ( a ) Schematic representation of the maternal and paternal genomic regions in which the miR-371-3 locus resides. Filled circle: methylated allele; empty circle: unmethylated allele. Maternally expressed genes and PEGs are designated in red and blue, respectively. Genes with biallelic expression are shown in grey. Note that current data regarding the parental expression of ZNF331 are conflicting. ( b ) Mean methylation calls±s.d. across the region in different cell types; WT-HESCs ( n =20), WT-HiPSCs ( n =12), WT-Fib ( n =6), PgHiPSCs ( n =4) and Pg-Fib ( n =2). DNA methylation levels ( y -axis) vary between 0 (unmethylated) and 1 (fully methylated); 0.4–0.6, intermediate methylation values. ( c ) Expression levels (mean±s.d., in two WT-PSC lines and three PgHiPSC lines) of all annotated miRs in the region in WT-HiPSCs and PgHiPSCs. ( d ) Expression levels (mean±s.d., in two WT-PSC lines and two PgHiPSC lines) of annotated genes within the region, as determined by RNA sequencing analysis. Full size image A functional link between anti-miR-371-3 and miR-371-3 To examine a possible functional link between anti-miR-371-3 and its corresponding miRs, we asked whether the upregulation of miR-371-3 in PgHiPSCs results from downregulation of anti-miR-371-3 in these cells. We therefore specifically knocked down anti-miR-371-3 in normal HiPSCs ( Fig. 3a ), followed by quantitative real-time (qRT)–PCR for analysis of miR-371-3 expression ( Fig. 3b ). Our results show that inhibition of anti-miR-371-3 leads to upregulation of miR-371-3 in normal cells to an extent comparable with PgHiPSCs, suggesting that anti-miR-371-3 directly regulates the expression of the corresponding miRs ( Fig. 3a,b ). Subsequently, we hypothesized that the expression of anti-miR-371-3 may be regulated by the regional imprinted DMR upstream to ZNF331 or, alternatively, by currently unidentified DMR. Specifically, anti-miR-371-3 may appear downregulated in parthenogenetic cells because of hypermethylation of this putative DMR, similar to other known PEGs. We thus aimed to remove the inhibition of anti-miR-371-3 in PgHiPSCs by treatment with 5-azacytidine, a known demethylating agent [20] . Interestingly, following 3 days of treatment with 5-azacytidine at a low concentration (0.5 μM), detectable expression levels of anti-miR-371-3 were observed, resulting in downregulation of the corresponding miRs ( Fig. 3c ). This treatment, however, had no significant effect on the expression of either transcript in normal PSCs, probably because of the relatively low sensitivity of our methodology to detect small changes in the expression of both strands ( Fig. 3c ). To exclude the possibility that 5-azacytidine may affect miR-371-3 independently of anti-miR-371, we treated PgHiPSCs with 5-azacytidine while specifically knocking down anti-miR-371-3. In contrast to treatment with 5-azacytidine alone, simultaneous inhibition of anti-miR-371-3 prevents the downregulation of miR-371-3 ( Fig. 3c ). Moreover, treatment with 5-azacytidine resulted in a shift from monoallelic to biallelic expression of anti-miR-371 ( Fig. 3d ). Collectively, our results suggest that hypermethylation in PgHiPSCs, leading to loss-of-imprinting of anti-miR-371-3, facilitates the overexpression of miR-371-3 in these cells. 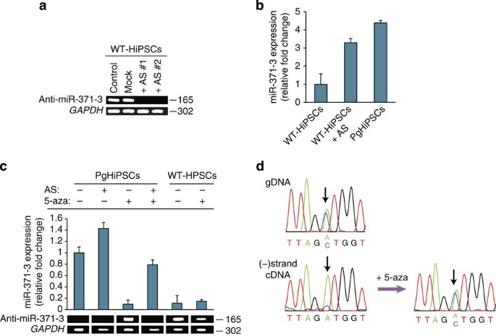Figure 3: Effects of anti-miR-371-3 inhibition on the expression of miR-371-3. (a) Strand-specific RT-PCR of anti-miR-371-3 following its inhibition in normal PSCs using an antisense of anti-miR-371-3 (AS). Shown are two clones treated with AS. (b) Relative expression levels of miR-371-3 (mean±s.d.) in normal PSCs before and after inhibition of anti-miR-371-3, relative to PgHiPSCs, as analysed by qRT–PCR. Shown is the mean level measured in the two clones treated with AS. (c) Strand-specific RT–PCR for detection of anti-miR-371-3 in PgHiPSCs (lower inset, band sizes are designated in bp), and the relative expression levels of miR-371-3 (mean±s.d. in two PgHiPSC lines, upper inset) as analysed by qRT–PCR, following 72 h of treatment with 0.5 μM 5-azacytidine (5-aza), inhibition of anti-miR-371-3 (AS) or a combined treatment. Average expression in two normal PSCs was used as control. (d) Strand-specific sequencing of anti-miR-371-3 in a normal PSC line before and after demethylation. Shown is a heterozygous single nucleotide polymorphism in the genomic DNA (gDNA) and monoallelic expression of anti-miR-371-3. Biallelic expression of anti-miR-371-3 was evident following 72 h of treatment with 0.5 μM 5-azacytidine. Figure 3: Effects of anti-miR-371-3 inhibition on the expression of miR-371-3. ( a ) Strand-specific RT-PCR of anti-miR-371-3 following its inhibition in normal PSCs using an antisense of anti-miR-371-3 (AS). Shown are two clones treated with AS. ( b ) Relative expression levels of miR-371-3 (mean±s.d.) in normal PSCs before and after inhibition of anti-miR-371-3, relative to PgHiPSCs, as analysed by qRT–PCR. Shown is the mean level measured in the two clones treated with AS. ( c ) Strand-specific RT–PCR for detection of anti-miR-371-3 in PgHiPSCs (lower inset, band sizes are designated in bp), and the relative expression levels of miR-371-3 (mean±s.d. in two PgHiPSC lines, upper inset) as analysed by qRT–PCR, following 72 h of treatment with 0.5 μM 5-azacytidine (5-aza), inhibition of anti-miR-371-3 (AS) or a combined treatment. Average expression in two normal PSCs was used as control. ( d ) Strand-specific sequencing of anti-miR-371-3 in a normal PSC line before and after demethylation. Shown is a heterozygous single nucleotide polymorphism in the genomic DNA (gDNA) and monoallelic expression of anti-miR-371-3. Biallelic expression of anti-miR-371-3 was evident following 72 h of treatment with 0.5 μM 5-azacytidine. Full size image Involvement of anti-miR-371-3 in TGCTs An accumulating body of work links the overexpression of miR-372-3 with cell proliferation in different types of tumours [9] , [21] , [22] . Particularly, an oncogenic role for miR-372-3 was previously recognized in TGCTs where these miRs were shown to contribute to proliferation and cellular transformation [9] . This is of special interest as germ cell tumours feature expression patterns resembling those of PSCs [23] , whose unique miR-371-3 expression signature [11] was recently associated with cellular reprogramming [24] and differentiation potential [25] . We thus hypothesized that similar to PgHiPSCs, TGCTs expressing high levels of miR-371-3 might have lost the imprint of the corresponding anti-miR-371-3. We therefore analysed a TGCT cell line exhibiting high expression levels of miR-371-3 (Tera1) [9] . As a control, we also studied an embryonal carcinoma cell line (NTera2) that exhibits a pluripotent signature, thereby predicted to express both transcripts. Studying the expression profiles of anti-miR-371-3 pointed to inhibition of this transcript in Tera1, but not in NTera2 cells ( Fig. 4a ), oppositely correlating with the differential expression of miR-371-3 in these cells ( Supplementary Fig. S1d ). Next, we examined whether global demethylation would affect the expression of anti-miR-371-3 in Tera1 cells similar to parthenogenetic cells. We therefore treated Tera1 cells with 5-azacytidine and examined its effect on both sense and antisense transcripts. Following 3 days of treatment with 2 μM of 5-azacytidine, we could document notable expression levels of anti-miR-371-3 and consequently significant downregulation of miR-371-3 ( Fig. 4b ). As in PgHiPSCs, the effect on the miR-371-3 locus was specific, as simultaneous treatment with both 5-azacytidine and inhibitor of anti-miR-371-3 did not affect miR-371-3 expression ( Fig. 4b ). As miR-372-3 were shown to have an oncogenic role in several types of cancers, we speculated that their newly identified antisense transcript may hold a tumour suppressive potential. To study the effect of anti-miR-371-3 on cell growth, we sought to introduce it into Tera1 cells. To this end, we generated two expression constructs, one spanning the promoter region and miR-371-3 transcript and a truncated version that does not overlap the promoter region ( Fig. 4c ). Following transfection of Tera1 cells with each construct, detectable levels of anti-miR-371-3 were observed, consequently leading to downregulation of miR-371-3 ( Fig. 4d ). Interestingly, a major reduction in cell number was observed in the anti-miR-371-3-overexpressing cells compared with control cells ( Fig. 4e ). This phenotype was recapitulated in Tera1 cells expressing the truncated construct, demonstrating that the overlap between the transcripts is sufficient for miR-371-3 regulation ( Supplementary Fig. S1e ). Next, we monitored cell growth following introduction of anti-miR-371-3. Our results demonstrate significant reduction in the number of anti-miR-371-3-overexpressing cells relative to control cells ( Fig. 4f ). This effect was partially rescued by simultaneously overexpressing the miR-371-3 cluster and anti-miR-371-3 ( Fig. 4f ). Alternatively, treatment with 5-azacytidine recapitulated the phenotype of cell growth arrest in Tera1 cells ( Fig. 4g ). 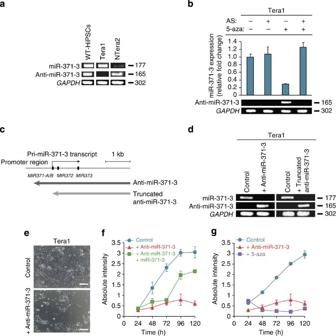Figure 4: Involvement of anti-miR-371-3 in TGCTs. (a) Strand-specific RT–PCR of miR-371-3 and anti-miR-371-3 in different cell lines. Band sizes are designated in bp. (b) Strand-specific RT-PCR for detection of anti-miR-371-3 in Tera1 cells (lower inset, band sizes are designated in bp), and the relative expression levels of miR-371-3 (mean±s.d. in four biological replicates, upper inset) as analysed by qRT–PCR, following 72 h of treatment with 2 μM 5-azacytidine (5-aza), inhibition of anti-miR-371-3 (AS) or a combined treatment. (c) Schematic diagram of the anti-miR-371-3 overexpression constructs in respect to the miR-371-3 locus. (d) Strand-specific RT-PCR of miR-371-3 and anti-miR-371-3 in Tera1 cells following transfection with each of the anti-miR-371-3 overexpression constructs. Band sizes are designated in bp. (e) Significant reduction in Tera1 cell number was observed 72 h following transfection with the anti-miR-371-3 overexpression construct (lower inset), as compared with control cells transfected with an empty vector (upper inset); scale bar=200 μm. (f–g) Viability assays of Tera1 cells, as measured by methylene blue staining (mean±s.d.,n=4). (f) Tera1 cells were treated with an empty vector (blue), with anti-miR-371-3 expression vector (red) or with a combination of miR-371-3 and anti-miR-371-3 expression vectors (green). (g) Tera1 cells were treated with an empty vector (blue), with anti-miR-371-3 expression vector (red) or with 2 μM 5-azacytidine (5-aza) (purple). Figure 4: Involvement of anti-miR-371-3 in TGCTs. ( a ) Strand-specific RT–PCR of miR-371-3 and anti-miR-371-3 in different cell lines. Band sizes are designated in bp. ( b ) Strand-specific RT-PCR for detection of anti-miR-371-3 in Tera1 cells (lower inset, band sizes are designated in bp), and the relative expression levels of miR-371-3 (mean±s.d. in four biological replicates, upper inset) as analysed by qRT–PCR, following 72 h of treatment with 2 μM 5-azacytidine (5-aza), inhibition of anti-miR-371-3 (AS) or a combined treatment. ( c ) Schematic diagram of the anti-miR-371-3 overexpression constructs in respect to the miR-371-3 locus. ( d ) Strand-specific RT-PCR of miR-371-3 and anti-miR-371-3 in Tera1 cells following transfection with each of the anti-miR-371-3 overexpression constructs. Band sizes are designated in bp. ( e ) Significant reduction in Tera1 cell number was observed 72 h following transfection with the anti-miR-371-3 overexpression construct (lower inset), as compared with control cells transfected with an empty vector (upper inset); scale bar=200 μm. ( f – g ) Viability assays of Tera1 cells, as measured by methylene blue staining (mean±s.d., n =4). ( f ) Tera1 cells were treated with an empty vector (blue), with anti-miR-371-3 expression vector (red) or with a combination of miR-371-3 and anti-miR-371-3 expression vectors (green). ( g ) Tera1 cells were treated with an empty vector (blue), with anti-miR-371-3 expression vector (red) or with 2 μM 5-azacytidine (5-aza) (purple). Full size image Anti-miR-371-3 has a tumour suppressive role in TGCTs To evaluate the pathway in which anti-miR-371-3 overexpression affects the proliferation of Tera1 cells, we stained both control and anti-miR-371-3-overexpressing cells with an antibody against annexin-V, a known marker for cellular apoptosis. Flow cytometry analysis demonstrated significantly higher levels of cellular apoptosis in anti-miR-371-3-overexpressing cells (32% compared with 2.9% in control cells; Fig. 5a ). Next, we examined the effect of anti-miR-371-3 on cell cycle. Our results indicate that anti-miR-371-3-overexpressing cells accumulate in the G2/M stage ( Fig. 5b ). These findings are in agreement with a previous report [21] , by which specific inhibition of miR-372-3 in human gastric cancer cell lines results in cell cycle arrest in the G2/M stage, along with increased levels of cellular apoptosis. To test the ability of anti-miR-371-3 to inhibit tumour formation in vivo , Tera1 cells were infected with lentiviruses carrying either anti-miR-371-3 or an empty control vector. Following 48 h, three million cells from each treatment were injected subcutaneously to immunodeficient mice. Correspondingly, similar numbers of cells were replated and kept under standard conditions to monitor cell growth in vitro . A significant reduction in the number of cells overexpressing anti-miR-371-3 was documented after 48 h. This phenotype coincided with changes in the morphology of the cells, which became flattened and ceased to proliferate in culture over the course of 2 weeks. As expected, during a period of 5–6 weeks after injection, tumours were documented in the control cells. On the other hand, in Tera1 cells overexpressing anti-miR-371-3 tumour formation was completely inhibited ( Fig. 5c and Table 1 ). Therefore, we suggest that anti-miR-371-3 has a tumour suppressive role in TGCTs, as its overexpression in cancer cells prevents tumour formation in vivo . A well-established target of miR-372-3 is the large tumour suppressor homologue 2 ( LATS2 ) [9] , [21] , whose deletion in mice was previously shown to increase cell proliferation and tumour development [26] . We thus inferred that overexpression of anti-miR-371-3 in Tera1 cells should remove LATS2 inhibition by miR-372-3 and result in cell growth arrest. Analysing expression levels of LATS2 in anti-miR-371-3-overexpressing Tera1 cells demonstrated a significant upregulation relative to control cells ( Fig. 6a and Supplementary Fig. S1f ). The miR-371-3 cluster is predicted to regulate expression of additional genes other than LATS2 , some of which may contribute to tumorigenicity [24] . To study whether LATS2 has a key role in suppressing cell growth, subsequently to activation of anti-miR-371-3, we simultaneously overexpressed anti-miR-371-3 while knocking down LATS2 in Tera1 cells ( Fig. 6a and Supplementary Fig. S1g ). Remarkably, downregulation of LATS2 allowed the cells to bypass the anti-miR-371-3-mediated growth inhibition ( Fig. 6b ). 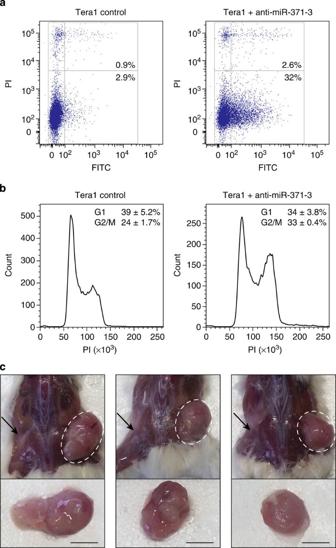Figure 5: A potential tumour suppressive role of anti-miR-371-3 in TGCTs. (a) Apoptosis analysis in anti-miR-371-3-overexpressing Tera1 cells (right panel) and untreated Tera1 cells (left panel). Right lower gate represents annexin-V-positive cells (32% and 2.9%, respectively). (b) Cell cycle analysis demonstrating accumulation of anti-miR-371-3-overexpressing Tera1 cells in the G2/M stage. Shown are mean values±s.d. (n=3). (c) Tera1 cells were infected with lentiviruses carrying either the anti-miR-371-3 construct or an empty vector as control. Approximately 3 × 106cells were injected subcutaneously to immunodeficient mice. Five to six weeks after injection, tumours were documented in control cells (dashed circle and lower panel), whereas Tera1 overexpressing anti-miR-371-3 did not generate tumours (black arrows). Scale bar, 1 cm. Figure 5: A potential tumour suppressive role of anti-miR-371-3 in TGCTs. ( a ) Apoptosis analysis in anti-miR-371-3-overexpressing Tera1 cells (right panel) and untreated Tera1 cells (left panel). Right lower gate represents annexin-V-positive cells (32% and 2.9%, respectively). ( b ) Cell cycle analysis demonstrating accumulation of anti-miR-371-3-overexpressing Tera1 cells in the G2/M stage. Shown are mean values±s.d. ( n =3). ( c ) Tera1 cells were infected with lentiviruses carrying either the anti-miR-371-3 construct or an empty vector as control. Approximately 3 × 10 6 cells were injected subcutaneously to immunodeficient mice. Five to six weeks after injection, tumours were documented in control cells (dashed circle and lower panel), whereas Tera1 overexpressing anti-miR-371-3 did not generate tumours (black arrows). Scale bar, 1 cm. Full size image Table 1 Summary of in vivo tumour formation. 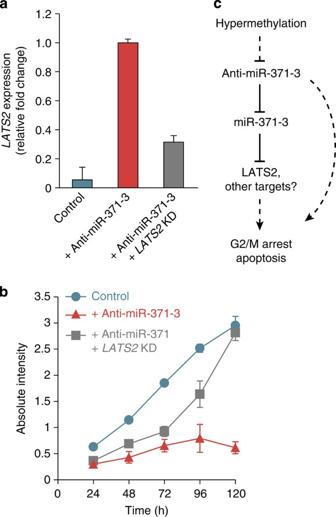Figure 6:LATS2is a downstream target of anti-miR-371-3. (a) The effect ofLATS2knockdown in Tera1 cells overexpressing anti-miR-371-3. Relative expression levels ofLATS2were analysed by qRT–PCR 72 h after transfections (mean±s.d. in three biological replicates). (b) Viability assay of Tera1, measured by methylene blue staining (mean±s.d.,n=3). (c) Schematic model of the mechanism by which downregulation of anti-miR-371-3 may contribute to an oncogenic pathway in TGCTs. Full size table Figure 6: LATS2 is a downstream target of anti-miR-371-3. ( a ) The effect of LATS2 knockdown in Tera1 cells overexpressing anti-miR-371-3. Relative expression levels of LATS2 were analysed by qRT–PCR 72 h after transfections (mean±s.d. in three biological replicates). ( b ) Viability assay of Tera1, measured by methylene blue staining (mean±s.d., n =3). ( c ) Schematic model of the mechanism by which downregulation of anti-miR-371-3 may contribute to an oncogenic pathway in TGCTs. Full size image Emerging evidence links miR-372-3 with cell proliferation and tumorigenicity in different cancers. Here we report that these onco-miRs are tightly regulated by an imprinted antisense transcript. Interestingly, previous studies in flies and mice revealed that distinct sense and antisense miRs can be generated from transcription of the same hairpin region in opposite orientations [27] , [28] . Our data indicate that the overlap region between anti-miR-371-3 and the corresponding miR transcripts is sufficient to inhibit the expression of miR-371-3. It will therefore be of interest to elucidate whether anti-miR-371-3 is further processed into endogenous mature miRs, potentially regulating additional downstream targets other than miR-372-3. The intrinsic monoallelic nature of anti-miR-371-3, which renders it highly susceptible to alterations, is of particular importance. Our comprehensive DNA methylation analysis of the miR-371-3 region could verify a previously proposed imprinted maternal DMR, suggesting that similar to other imprinted loci, it may regulate the parent-of-origin expression of multiple genes in its proximity. Supporting this notion, we suggest that a hypermethylation event leading to loss-of-imprinting of anti-miR-371-3 accounts for the upregulation of miR-371-3 in parthenogenesis and TGCTs ( Fig. 6c ). To study the role of anti-miR-371-3 in TGCTs, we reintroduced it into Tera1 cells and demonstrated marked effects on cell proliferation, in coincidence with cell growth arrest and apoptosis ( Fig. 6c ). Further, overexpression of anti-miR-371-3 completely inhibited tumour formation in vivo , suggesting that this novel imprinted transcript has a tumour suppressive role in TGCTs. Our analysis to examine the effect of anti-miR-371-3 on its putative downstream targets pointed to a pivotal role of LATS2 in enhancing cell growth arrest. Nevertheless, this does not preclude the involvement of other potential targets, either directly or indirectly regulated by anti-miR-371-3 and miR-371-3 ( Fig. 6c ). Previous studies have emphasized the unique expression pattern of miR-371-3 in PSCs [11] , [24] , which was also shown to predict their neuronal differentiation potential [25] . It would thus be valuable to study the interplay between miR-371-3 and their antisense transcript during early development. Reciprocal regulation of this kind is likely, given the perfect complementarity between the transcripts. In support of this possibility, miRs in the imprinted Dlk1-Dio3 region were previously shown to control the abundance of their antisense Rtl1 gene [29] . Finally, despite the inherent monoallelic nature of imprinted genes, only little is known about their involvement in tumorigenic progression. Our study sheds light on the contribution of loss-of-imprinting of a novel PEG to cell proliferation and tumorigenicity in TGCTs, with potential implications for future cancer therapy. Cell culture Normal and parthenogenetic PSC cultures were maintained on mitomycin-arrested mouse embryonic fibroblasts feeder layer and were grown in HESC medium containing Knockout Dulbecco’s Modified Eagle’s Medium (Gibco) supplemented with 15% Knockout Serum Replacement (Gibco), 2 mM L -glutamine (Biological Industries, Israel), 0.1 mM nonessential amino acids (Biological Industries), 0.1 mM β-mercaptoethanol and 8 ng ml −1 basic fibroblast growth facactor (Cytolab). All cells were maintained in a humidified incubator at 37 °C and 5% CO 2 . PSCs were collected using trypsin (Biological Industries). Tera1 cells were cultured in McCoy’s 5A medium modified (Sigma-Aldrich), supplemented with 15% fetal calf serum (Biological Industries), 2 mM L -glutamine (Biological Industries), 50 units per ml of penicillin and 50 μg ml −1 streptomycin (Biological Industries). Differentiation of human PSCs Trophectoderm-like cells derived from human PSCs were established as previously described [10] . NCAM1-positive cells were derived from human PSCs using a previously reported protocol for direct neural differentiation [30] with slight modification. Briefly, PSC colonies were cultured as EBs for 4 days in DMEM-F12 medium (Sigma-Aldrich) supplemented with 15% Knockout Serum Replacement (Gibco), 2 mM L -glutamine (Biological Industries), 0.1 mM nonessential amino acids (Biological Industries), 0.1 mM β-mercaptoethanol, 50 units per ml penicillin, 50 μg ml −1 streptomycin, 5 μM dorsomorphin (Tocris Bioscience) and 5 μM SB431542 (Cayman Chemical). EBs were then plated for neural expansion on 0.2% gelatin-coated plates and cultured for additional 6 days in DMEM-F12 medium supplemented with 1 × N2 (Gibco), 2 mM L -glutamine and 20 ng ml −1 basic fibroblast growth factor (Cytolab). Neural cells expressing NCAM1 were sorted by flow cytometry using hNCAM-1/CD56 antibody (1:150, R&D). miRNA expression analysis Total RNA was extracted using MirVana miRNA isolation kit (Ambion Inc). RNA was subjected to Human GeneChip miRNA array platform (Affymetrix, CA), according to the manufacturer’s protocol. Data were normalized using miRNA QC Tool (Affymetrix). High-throughput sequencing Total RNA was extracted using MirVana miRNA isolation kit (Ambion Inc) according to the manufacturer’s protocol. Libraries were generated following ribosomal RNA depletion (RiboMinus, Invitrogen). The SOLiD (version 3.5) sequencing technology (Life Technologies) was used to generate 35-bp-long reads, which were aligned to UCSC complete build (GRCh37/hg19) genome. Reads that mapped to contaminants such as transfer RNA, ribosomal RNA and DNA repeats were filtered out. Sequences for each transcript were calculated in RPKM (reads per kilobase of exon model per million mapped reads) units using TopHat/Cufflinks combination to obtain normalization of the number of reads relative to their transcript length. Each region was then assigned with a value of false discovery rate. Subsequently, to lower the possibility of false detection, regions with minimal threshold of RPKM expression (that is, false discovery rate P -value >0.05) were filtered out. The P -value for differential gene expression between samples was calculated for expressed genes only. Significant differences were considered for P <0.05. The high-throughput data were deposited in the GEO database (Accession code: GSE47088). DNA methylation analysis Reduced representation bisulphite sequencing libraries were generated according to standard procedures [31] , [32] . The bioinformatic analysis was performed as previously described [15] , [32] . In brief, to study DNA methylation signature throughout the miR-371-3 locus, weighted average methylation values were calculated for each region and for each cell line included in the study. Mean methylation value for each region was calculated for all cell lines of the same cell type (for example, HESCs, HiPSCs, WT-Fib and so on). To identify putative imprinted DMRs, we searched for intermediately methylated regions in both HESCs and HiPSCs and compared them to the methylation values of the parthenogenetic samples (regions in which the difference between PgHiPSCs and HESCs was lower than 0.2 were filtered out). Isolation of genomic DNA and RNA and reverse transcription Total genomic DNA was extracted using Nucleic Acid and Protein Purification kit (Macherey-Nagel Corporation) and RNA (DNase treated) was purified with PerfectPure RNA Cultured Cell kit (5-Prime). One microgram of total RNA was used for reverse transcription using ImProm-II reverse transcriptase (Promega) with random hexamer primers. For strand-specific reverse transcription a single primer was used, corresponding either to the positive or negative strands (20 μM). For sequencing and quantitative experiments, PCR was performed with GoTaq (Promega), whereas for overexpression experiments PCR reactions Platinum Pfx DNA Polymerase (Invitrogen) was used. qRT–PCR was performed with 1 μg of RNA reverse transcribed to complementary DNA and TaqMan Universal Master Mix or SYBR green qPCR Supermix. Data were analysed with the 7300 real-time–PCR system (Applied Biosystems). A full description of primer sequences and annealing temperature are found in Supplementary Table S1 . Manipulation of anti-miR-371-3 in PgHiPSCs and Tera1 cells For specific inhibition of anti-miR-371-3, a combination of four single-stranded DNA molecules (primers are described in Supplementary Table S1 ) were co-transfected into Tera1 cells using Lipofectamine 2000 reagent (Invitrogen), according to the manufacturer’s instructions. Demethylation experiments were performed using 5-azacytidine (Sigma). Fresh medium supplemented with 5-azacytidine was supplied to PgHiPSCs (0.5 μM) and Tera1 cell (2 μM) every other day. For overexpression experiments, anti-miR-371-3 or anti-miR-371-3-truncated sequences were amplified by PCR (primers are described in Supplementary Table S1 ) and cloned into an N1-EGFP vector using DNA Ligation Kit (Mighty Mix, TaKaRa). For experiments involving overexpression, we used both TransIT-LT1 (Mirus) transfection reagent and electroporation (Gene Pulser Xcell, Bio-Rad, 300 V, 500 μF, 4 mm cuvette) to transiently transfect Tera1 cells. In each case, 15 μg of plasmid DNA were used. Overexpression of miR-371-3 cluster (kindly donated by Professor Reuven Agami [9] ) was performed using TransIT-LT1 (Mirus) transfection reagent, according to the manufacturer’s instructions. Knockdown of LATS2 in HEK-293T and Tera1 cells For short interfering RNA transfection, HEK-293T and Tera1 cells were dissociated using 0.25% trypsin EDTA solution (Biological Industries), counted and replated at 1 × 10 6 cells per well on a six-well plate (HEK-293T cells) or at 1 × 10 5 cells per well in a 24-well plate (Tera1 cells). On the following day, cells were transected with 10 or 2 μl, respectively, of 20 μM ON-Target-Plus smart pool siRNA (Thermo Scientific) using Lipofectamine2000 reagent (Life technologies) according to the manufacturer’s instructions. Cells were collected for RNA extraction 48 and 72 h after transfection. Cell viability assay Methylene blue assay was used to quantify the relative number of cells following different treatments of Tera1. Cells were fixated with 0.5% glutardialdehyde (Sigma-Aldrich) and stained with methylene blue (Sigma-Aldrich) dissolved in 0.1 M boric acid (pH 8.5). Colour extraction was performed using 0.1 M hydrochloric acid and quantified by measuring absorbance at 650 nm. Flow cytometry Tera1 cells were dissociated using Tripleselect (Gibco) and washed with FACS medium (PBS containing 10% fetal calf serum). For detection of cellular apoptosis, Annexin-V staining was performed using annexin-V kit (Bender MedSystems, Burlingame, CA) according to the manufacturer’s instructions. For cell cycle analysis, Tera1 cells were dissociated using trypsin EDTA solution B (Biological Industries), resuspended in cold 100% methanol and kept for at least 2 h at −20 ° C. Cells were then washed and resuspended in PBS containing 0.2 μg μl −1 RNAse for 0.5 h. Propidium iodide was added to the cells to a final concentration of 50 μg ml −1 for 5 min. Experiments were performed on FACSaria system (Becton, Dickinson and Company, Franklin Lakes, NJ). Analysis was performed using FlowJo software (TREE STAR, Inc.). Tumour formation experiments All experimental procedures were approved by the ethics committee of the Hebrew University. For in vivo experiments, the sequence of anti-miR-371-3 was amplified by PCR (primers are described in Supplementary Table S1 ) and cloned into a pLVGUS-DsRed lentiviral vector using DNA Ligation Kit (Mighty Mix, TaKaRa). For production of lentiviral particles, 2 × 10 6 HEK-293T cells in a 10-cm dish were transfected using TransIT-LT1 (Mirus) with 6.25 μg of the target vector, 2.18 μg of pCMV-VSV-G and 4.08 μg of gag/pol plasmid (Addgene). Forty-eight and 72 h after transfection, the supernatant was collected, filtered through a 0.45-μM cellulose acetate filter (Whatman) and supplemented with 4 μg ml −1 of Polybrene (Sigma-Aldrich). Approximately 3 × 10 6 Tera1 cells were infected with lentiviral particles containing either the anti-miR-371-3 overexpression construct or an empty pLVGUS-DsRed vector for control. Three days after transfection, Tera1 cells were dissociated and injected subcutaneously to male immunodeficient mice (7–9 weeks of age; Jackson Laboratory). Five to six weeks after injection, mice were killed and tumours were dissected and analysed. Accession codes: The high-throughput sequencing data have been deposited in the GEO database under Accession code GSE47088 . How to cite this article: Stelzer, Y. et al. Involvement of parental imprinting in the antisense regulation of onco-miR-372-373. Nat. Commun. 4:2724 doi: 10.1038/ncomms3724 (2013).